Integration of Hippo signalling and the unfolded protein response to restrain liver overgrowth and tumorigenesis The role of the unfolded protein response (UPR) in tissue homeostasis remains largely unknown. Here we find that loss of Mst1/2, the mammalian Hippo orthologues, or their regulator WW45, leads to a remarkably enlarged endoplasmic reticulum (ER) size-associated UPR. Intriguingly, attenuation of the UPR by tauroursodeoxycholic acid (TUDCA) diminishes Mst1/2 mutant-driven liver overgrowth and tumorigenesis by promoting nuclear exit and degradation of Hippo downstream effector Yap. Yap is required for UPR activity and ER expansion to alleviate ER stress. During the adaptive stage of the UPR, PERK kinase-eIF2α axis activates Yap, while prolonged ER stress-induced Hippo signalling triggers assembly of the GADD34/PP1 complex in a negative feedback loop to inhibit Yap and promote apoptosis. Significantly, the deregulation of UPR signals associated with Yap activation is found in a substantial fraction of human hepatocellular carcinoma (HCC). Thus, we conclude Yap integrates Hippo and UPR signalling to control liver size and tumorigenesis. The endoplasmic reticulum (ER) is the primary subcellular organelle responsible for protein folding, the biosynthesis of lipids and sterols, and calcium storage in eukaryotic cells. Alterations in ER homeostasis lead to the accumulation of unfolded or misfolded proteins in the ER lumen, which is referred to as ER stress. In cells experiencing ER stress, activation of the unfolded protein response (UPR) reduces unfolded/misfolded protein loads through diverse pro-survival mechanisms, such as the expansion of the ER membrane, the attenuation of general protein synthesis and the selective synthesis of key components of the protein folding and quality control machinery in the ER. However, a failure to restore ER homeostasis by the UPR leads to the initiation of pro-apoptotic pathways in cells [1] , [2] . Remarkably, UPR dysregulation has been implicated in many human diseases, including diabetes, cardiovascular diseases, neurodegenerative diseases, viral infections and cancers [3] . Different ER stress transducers located on the ER membrane, such as PKR-like ER kinase (PERK), inositol-requiring enzyme 1 (IRE1) and activating transcription factor 6 (ATF6), can initiate distinct UPR signalling pathways. In the absence of stress, all ER stress transducers are sequestered by the ER HSP70 family protein Bip (GRP78; HSPA5). The competitive binding of Bip by the hydrophobic surfaces of misfolded proteins following ER stress releases these transducers to trigger UPR signalling. However, the mechanisms underlying the stress-specific activation of selected UPR signalling in the determination of cell fate is unclear [2] . Eukaryotic initiation factor 2α (eIF2α), which is a critical component in the formation of the translation initiation ternary complex (eIF2α/GTP/methionyl transfer RNA), plays a key role in the ER stress response [4] . During the adaptive stage of ER stress, the phosphorylation of eIF2α at serine 51 by PERK suppresses general protein synthesis and specifically induces the translation of ATF4 to promote cell survival [5] . PERK-eIF2α-ATF4 pathway is required not only for translational control, but also necessary for ATF6 cleavage and subsequent activation. X-box binding protein 1 (Xbp1) messenger RNA is induced by ATF6 and spliced by IRE1 in response to ER stress, to produce a highly active transcription factor (Xbp1s), which is critical for cell fate determination in response to ER stress [6] . In addition, prolonged ER stress induces the transcription of C/EBP homologous protein (CHOP, Ddit3) and growth arrest and DNA damage-inducible protein 34 (GADD34) via ATF4 (ref. 7 ). ATF4 and CHOP can act together to restore general mRNA translation, leading to cell death [8] . Moreover, GADD34 and its structural homologue, the constitutive repressor of eIF2α phosphorylation (CReP), assemble protein phosphatase 1 (PP1), which functions in a negative feedback loop to dephosphorylate eIF2α and suppress the UPR to promote cell death [9] . However, the molecular mechanisms underlying the switch between the pro-survival and pro-apoptotic responses of the UPR remain unknown. The Hippo pathway is an evolutionarily conserved protein kinase cascade that negatively regulates the oncogenic transcriptional coactivator Yes-associated protein (Yap) and its paralogue, TAZ [10] , [11] , [12] , [13] . In the canonical Hippo pathway, the kinase core consists of the Ste20-like kinases Mst1/2 (Hippo in Drosophila ), which phosphorylate the nuclear Dbf2-related family kinases Lats1/2, and Mob1A/B in association with the WW-domain scaffolding protein WW45. Phospho-Mob1A/B activates Lats1/2 by inducing the autophosphorylation of Lats1/2, which in turn phosphorylate Yap to promote its binding to 14-3-3. The interaction with 14-3-3 causes Yap to exit from the nucleus, which inhibits its coactivator function. The dephosphorylation of Yap by PP1 results in its nuclear accumulation [14] , thereby promoting cell proliferation and inhibiting cell death via the TEAD transcription factor. Recent studies have shown that the Hippo pathway is regulated by cell architecture and mechanical signals [15] , [16] , [17] , and is involved in many membrane receptor signalling, including the G protein-coupled receptor [18] , epidermal growth factor receptor [19] and WNT receptor signalling [20] , [21] , [22] . We and others have found that the loss of any component of the Hippo core kinase cascade in mammals results in cell proliferation, resistance to apoptosis and massive organ overgrowth [23] , [24] , [25] , [26] , [27] , [28] , [29] , [30] . Similarly, the loss of Hippo signalling or the overexpression of a Hippo-resistant Yap mutant leads to the expansion of progenitor cells and cancer development in multiple organs [31] , [32] , [33] , [34] , [35] , [36] , [37] , [38] . Thus, the central function of the Hippo pathway is to inhibit the function of Yap, to restrain organ overgrowth [12] , [39] . Gene amplification of the Yap locus has been reported in a wide spectrum of human and murine malignancies [40] , [41] . We have previously shown that the Ets family transcriptional factor GABP is required for Yap expression [42] . Recently, verteporfin as a small molecule was shown to inhibit TEAD-Yap association and Yap-induced liver overgrowth [43] . Tauroursodeoxycholic acid (TUDCA), which is an endogenous bile acid (BA), is a well-known ER chaperone that alleviates ER stress, and it has shown therapeutic potential for treating diabetes and inflammation disease models [44] , [45] , [46] ; however, its underlying molecular mechanisms are poorly understood. Interestingly, in rat hepatocytes, TUDCA efficiently downregulates the expression of connective tissue growth factor (CTGF) [47] , which is a major target gene of Yap-TEAD, and CTGF is required for cell growth [48] . In this study, we found that TUDCA treatment hinders Mst1/2 mutant-driven liver overgrowth and tumorigenesis by promoting Yap nuclear exit and degradation. Further analyses reveal that the knockout of Mst1/2 or WW45 leads to elevated UPR signalling activities through Yap. By using biochemical and genetic approaches, we demonstrate that Hippo-Yap signalling restrains liver overgrowth and oncogenesis by modulating the UPR and ER size, and the disruption of these regulations has significant implications in human hepatocellular carcinoma (HCC) development and progression. Our data indicate that the inactivation of Hippo signalling in association with the upregulation of UPR signalling may be a general mechanism that drives liver cell malignant transformation. Yap may act as a switch between the pro-survival and pro-apoptotic responses of the UPR response. TUDCA retards Mst1/2 mutant-driven liver tumorigenesis Consistent with a previous report [47] , treatment with TUDCA, which is a hydrophilic BA derivative, downregulated the mRNA levels of the downstream Yap targets CTGF and Cyr61 in primary mouse hepatocytes ( Fig. 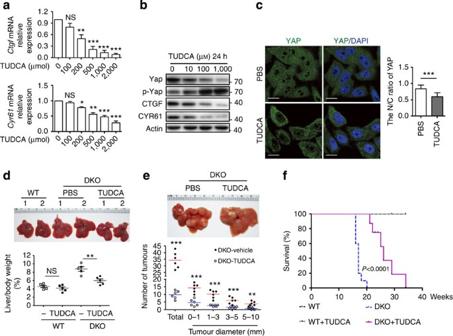Figure 1: TUDCA treatment inhibits Yap activation and abrogates Mst1/2 mutant-driven liver overgrowth and tumorigenesis. (a,b) Quantitative PCR analysis (a) or western blotting (b) showing the expression levels of CTGF, CYR61, phospho-Yap and total Yap in HepG2 cells following TUDCA treatment. (c) TUDCA treatment results in cytoplasmic retention of Yap in HepG2 cells. Yap subcellular localization was determined by immunofluorescence staining for endogenous Yap (green) along with DAPI for DNA (blue). Quantification of the ratio of nuclear (N) to cytoplasmic (C) Yap was shown in the right panel. Scale bar, 10 μm. (d–f) The liver sizes, liver-to-body weight ratios (d,n=5), sizes and numbers of liver tumours (e,n=6) and death ages (f,n=30) were significantly reduced in the TUDCA-treatedMst1−/−Mst2f/f-Abl-Cre(DKO) mice. The log-rank (Mantel–Cox) test,P<0.0001 (f). Data ina,d,ewere assessed by Student’st-test and represented as mean±s.d. ns, not significant, *P<0.05, **P<0.01, ***P<0.001 compared with respective controls or as indicated. Data are representative of at least three independent experiments. 1a and RNA sequencing (RNA-seq) data (NCBI GEO accession number GSE57654 ) in Supplementary Table 1 ). We further demonstrated that the TUDCA treatment inhibited Yap activity as shown by the increased Yap phosphorylation (Ser127) and its cytoplasmic retention, which thus decreased the expression of CTGF and CYR61 ( Fig. 1b,c and Supplementary Fig. 1a ). In addition, TUDCA treatment did not change the mRNA level of Yap, enhanced Yap ubiquitination, accelerated its degradation and decreased its protein levels ( Supplementary Fig. 1b–d ). Yap activation is critical in HCC development and in maintenance of Mst1 −/− Mst2 fl/fl Abl-Cre (double knockout (DKO)) mice [23] . Therefore, we examined whether TUDCA could attenuate HCC formation in DKO mice through the inhibition of Yap. Surprisingly, we found that the liver/body weight ratios were significantly decreased in 10-week-old DKO mice, which have been treated with 100 mg kg −1 TUDCA once a day for 2 weeks, while the sizes and numbers of tumours were also significantly decreased in 4-month-old mice, which have been treated with 250 mg kg −1 TUDCA twice per week for 2 months ( Fig. 1d,e ). The TUDCA treatment also delayed the death of the DKO mice ( Fig. 1f ). Moreover, the TUDCA treatment significantly decreased Yap nuclear localization and attenuated cell proliferation in the liver tissues of the DKO mice compared with those in the wild-type (WT) controls ( Supplementary Fig. 1d,e ). In addition, both short-term (2 weeks) and long-term (2 months) TUDCA treatments did not significantly change the tibial length of both WT and DKO mice. However, the long-term TUDCA treatment significantly increased the DKO mice body weight to the comparable levels of the WT mice treated with TUDCA ( Supplementary Fig. 2a–d ). Figure 1: TUDCA treatment inhibits Yap activation and abrogates Mst1/2 mutant-driven liver overgrowth and tumorigenesis. ( a , b ) Quantitative PCR analysis ( a ) or western blotting ( b ) showing the expression levels of CTGF, CYR61, phospho-Yap and total Yap in HepG2 cells following TUDCA treatment. ( c ) TUDCA treatment results in cytoplasmic retention of Yap in HepG2 cells. Yap subcellular localization was determined by immunofluorescence staining for endogenous Yap (green) along with DAPI for DNA (blue). Quantification of the ratio of nuclear (N) to cytoplasmic (C) Yap was shown in the right panel. Scale bar, 10 μm. ( d – f ) The liver sizes, liver-to-body weight ratios ( d , n =5), sizes and numbers of liver tumours ( e , n =6) and death ages ( f , n =30) were significantly reduced in the TUDCA-treated Mst1 −/− Mst2 f/f -Abl-Cre (DKO) mice. The log-rank (Mantel–Cox) test, P <0.0001 ( f ). Data in a , d , e were assessed by Student’s t -test and represented as mean±s.d. ns, not significant, * P <0.05, ** P <0.01, *** P <0.001 compared with respective controls or as indicated. Data are representative of at least three independent experiments. Full size image Hippo signalling controls UPR signalling and ER size in liver As a chemical chaperone, TUDCA alleviates ER stress [45] . Similar to TUDCA, another ER stress reducer, 4-phenylbutyric acid, also decreased Yap protein expression and activation ( Supplementary Fig. 2e ). Cellular adaptation to ER stress is achieved by the activation of UPR signalling. We therefore investigated whether the inactivation of Yap by TUDCA represents cross-talk between the Hippo and UPR signalling pathways. Interestingly, we found that the expression levels of the ER chaperone Bip as well as PERK and ATF6 branches of UPR signalling, including phospho-eIF2α, ATF4 and cleavaged ATF6 (ATF6(N)), were markedly enhanced in the primary hepatocytes or liver tissues of the DKO mice compared with WT controls, with the exception of both phospho-IRE1α level, and the ratio of Xbp1s/total Xbp1 were greatly reduced, indicating IRE1α activity is inhibited on the loss of Hippo signalling, although the total mRNA level of Xbp1 is increased in DKO samples ( Fig. 2a and Supplementary Fig. 3a–d ). In addition, transmission electron micrographs (TEMs) showed the remarkable enlargement of the ER compartments in the DKO hepatocytes ( Fig. 2b ). Similar results were found in the livers of the WW45 knockout mice ( Fig. 2c,d and Supplementary Fig. 3e ). Regarding the possibility that increased ER size or ER stress is just due to the increased proliferation mediated by the loss of tumour suppressors Mst1/2 or WW45, we examined another tumour suppressor gene p53 -deficient liver, which also develops liver tumours in a significant number of mice within 12 months [49] , and found that the p53 -deficient liver tissue exhibited normal ER size as compared with WT control by TEM analysis ( Supplementary Fig. 3f ). 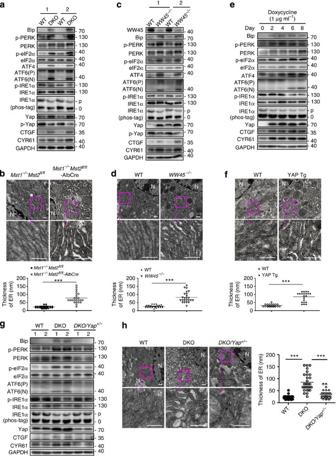Figure 2: Loss of function of the Hippo pathway results in a markedly elevated unfolded protein response in association with an enlarged ER size. Western blot analysis of UPR elements (a) and representative TEMs (b) of primary hepatocytes from WT and DKO mice. ER thickness was quantified for the indicated TEM samples. ATF6 (p) and (N), respectively, refer to ATF6 precursor and cleavaged form; IRE1α (p) and (0), respectively, refer to phospho- and non-phospho-IRE1α. The ‘N’ in TEMs refers to nuclear. Scale bar, 0.5 μm. (c,d) The assessment of UPR elements and ER sizes in the livers of WT andWW45f/f-Abl-Cre(WW45−/−) mice. Scale bar, 0.5 μm. (e,f) The assessment of UPR elements and ER sizes in the livers of WT and doxycycline-dependentYap (S127A)transgenic mice after 4-day oral administration of 1 μg ml−1doxycycline. Scale bar, 0.5 μm. (g,h) The assessment of UPR elements and ER sizes in the livers of WT, DKO andMst1−/−Mst2f/f-Yapf/+-Abl-Cre(DKO/Yap+/−) mice. Scale bar, 0.5 μm. Data were assessed by Student’st-test and represented as mean±s.d.n=24. ***P<0.001 compared with respective controls or as indicated. Figure 2: Loss of function of the Hippo pathway results in a markedly elevated unfolded protein response in association with an enlarged ER size. Western blot analysis of UPR elements ( a ) and representative TEMs ( b ) of primary hepatocytes from WT and DKO mice. ER thickness was quantified for the indicated TEM samples. ATF6 (p) and (N), respectively, refer to ATF6 precursor and cleavaged form; IRE1α (p) and (0), respectively, refer to phospho- and non-phospho-IRE1α. The ‘N’ in TEMs refers to nuclear. Scale bar, 0.5 μm. ( c , d ) The assessment of UPR elements and ER sizes in the livers of WT and WW45 f/f -Abl-Cre ( WW45 −/− ) mice. Scale bar, 0.5 μm. ( e , f ) The assessment of UPR elements and ER sizes in the livers of WT and doxycycline-dependent Yap (S127A) transgenic mice after 4-day oral administration of 1 μg ml −1 doxycycline. Scale bar, 0.5 μm. ( g , h ) The assessment of UPR elements and ER sizes in the livers of WT, DKO and Mst1 −/− Mst2 f/f -Yap f/+ -Abl-Cre (DKO/ Yap +/− ) mice. Scale bar, 0.5 μm. Data were assessed by Student’s t -test and represented as mean±s.d. n =24. *** P <0.001 compared with respective controls or as indicated. Full size image Reduced phospho-Yap levels and enhanced expression levels of CTGF and CYR61 were observed in both the DKO and WW45 KO livers, suggesting increased Yap activity ( Fig. 2a,c and Supplementary Fig. 3a,e ). Interestingly, the doxycycline-dependent induction of the Yap ( S127A ) transgene (an active form) dramatically enlarged ER sizes and increased UPR signalling in the livers after 4 days of doxycycline administration ( Fig. 2e,f and Supplementary Fig. 4a ). Moreover, TUDCA-treated DKO livers exhibited decreased ER size and attenuated UPR signalling, as shown by the lower levels of Bip and phospho-eIF2α, Yap, CTGF and higher level of phospho-Yap compared with the untreated controls ( Supplementary Fig. 4b,c ). To determine the effects of Yap on UPR signalling in the DKO livers, we analysed the expression levels of UPR elements in liver tissues from the WT, DKO or Mst1 −/− Mst2 f/f -Yap f/+ -Abl-Cre (DKO/Yap +/− ) mice. Comparable liver sizes, expression levels of Bip, phospho-PERK and phospho-eIF2α, and ER compartments were observed in the WT and DKO/Yap +/− mice, indicating that the deletion of only one Yap allele sufficiently attenuated UPR to its normal levels ( Fig. 2g,h and Supplementary Fig. 4d ), while no significant changed ER compartments were found in Yap −/− livers ( Supplementary Fig. 4e ). Taken together, these results suggest that Hippo/Yap signalling may have an important role in regulating UPR signalling and ER size. Yap regulates UPR signals and ER size through ATF6 To determine whether Yap can regulate UPR signalling and ER size in a cell-intrinsic manner, we generated the stable HepG2 cell lines with doxycline-induced overexpression or knockdown Yap. As expected, overexpression of Yap enhanced UPR signalling in HepG2 cells ( Fig. 3a and Supplementary Fig. 5a ). We next expressed a cytochrome β5-GFP fusion protein that allows for the visualization of ER compartments in HepG2 cells, and found that Yap knockdown reduced, whereas the overexpression of Yap enhanced, the appearance of morphologic changes in the ER, such as vacuolization and redistribution, which were triggered in response to treatment with 1 μg ml −1 of tunicamycin (TM), a pharmacological ER stress inducer that blocks the N -glycosylation of proteins ( Fig. 3b and Supplementary Fig. 5b ). We therefore speculate that Yap may be involved in the regulation of ER size in HepG2 cells. As expected, compared with the cells that were transfected with luciferase control vectors, the HepG2 cells overexpressing Yap exhibited the significantly enhanced fluorescence intensity of the ER-Tracker dye, indicating increased ER size expansion, regardless of the TM treatment. In contrast, Yap knockdown decreased the dye fluorescence intensity, indicating reduced ER sizes ( Fig. 3c ). Moreover, the TEMs confirmed that Yap knockdown slightly decreased basal ER sizes but completely blocked ER membrane expansion in the HepG2 cells during the TM-induced ER stress response ( Fig. 3d ). In addition, the overexpression of Yap enhanced, whereas its knockdown decreased, the ER Ca 2+ storage capabilities of the HepG2 cells ( Fig. 3e ). Although the knockdown of Yap slightly decreased basal mitochondrial sizes, as quantified by the Mito-Tracker dye, its overexpression did not significantly affect the mitochondrial sizes in the HepG2 cells regardless of the TM treatment ( Supplementary Fig. 5c ). Phosphorylation of IRE1α and Xbp1 mRNA splicing is the two common markers of the IRE1α branch activation of the UPR. Xbp1 has been linked to ER biogenesis and ER size expansion [50] , and recent study also showed that enforced expression of a constitutively active form of ATF6α trigger Xbp1-independent expansion of the ER [51] . We found that ATF6 but not IRE1α/Xbp1 is highly activated on the deletion of Mst1/2 or WW45 or overexpressing Yap transgene ( Fig. 2a,c,e and Supplementary Fig. 3c ). Activation of ATF6 requires cleavage first by a membrane-anchored serine protease (S1P) and subsequently by a membrane-embedded metalloprotease (S2P), to release the active transcription factor ATF6(N). Interestingly, the protein and/or RNA expression levels of proteases S2P, which might be responsible for increased ATF6(N), but not the S1P, were increased in the livers of both Mst1/2 DKO and Yap transgenic mice compared with those of their WT control ( Fig. 4a,b and Supplementary Fig 5d,e ). In addition, we found that TEAD could specifically bind to the S2P promoter in HepG2 cells using the chromatin immunoprecipitation assay ( Fig. 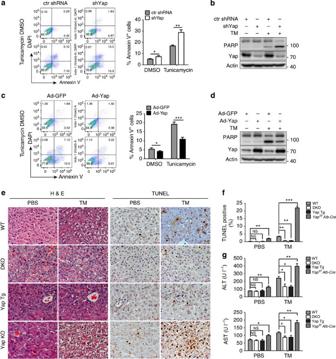Figure 5: Yap protects against ER stress-induced cell death and liver injury. Annexin V/DAPI staining and the cleavage of PARP in Yap knockdown (a,b) or overexpressing (c,d) HepG2 cells treated with 2 μg ml−1TM for 36 h. Bar graphs show the quantifications of Annexin V-positive cells in indicated samples,n=3. (e,f) Haematoxylin and eosin (H&E) or TUNEL staining of liver tissue sections from the WT,Mst1/2DKO,YapTg orYapfl/fl-Alb-Creknockout mice after a 3-day PBS or 0.5 mg kg−1TM treatment (e). Scale bar, 20 μm. Bar graphs show the quantifications of TUNEL-positive cells in the livers,n=5 (f). (g). Bar graphs show the quantifications of the serum ALT and AST levels of WT,Mst1/2DKO,YapTg orYapfl/fl-Alb-Cremice after 3-day PBS or 0.5 mg kg−1TM treatment. Data were assessed by Student’st-test and represented as mean±s.d. ns, not significant, *P<0.05, **P<0.01, ***P<0.001 compared with respective controls or as indicated. Data are representative of at least three independent experiments. 4c and Supplementary Fig. 5f ). Overexpression of Yap and/or TEAD enhanced the S2P promoter, but not TEAD-binding sites-mutated S2P promoter-driven luciferase activities ( Fig. 4d ). We then sought to determine the effect of ATF6 on Yap-mediated ER expansion. Indeed, knockdown of ATF6 significantly blocked the ER expansion induced by Yap, with or without TM treatment ( Fig. 4e ). 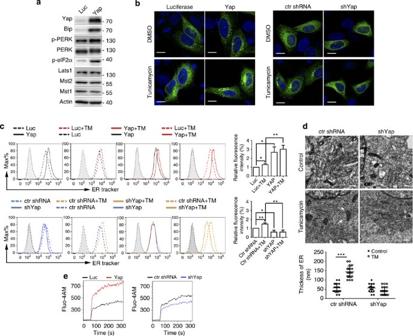Taken together, these results suggest that Yap regulates ER size and UPR activity through ATF6 branch of the UPR, to restore homeostasis during ER stress in a cell-intrinsic manner. Figure 3: Yap regulates UPR signalling and ER size in a cell-intrinsic manner. (a) Western blot analysis of UPR and Hippo signalling elements of HepG2 cells overexpressing luciferase or Yap. (b) The assessment of the role of Yap in the morphological changes of the ER (GFP fluorescence) in response to 1 μg ml−1TM treatment in HepG2 cells stably expressing cytochrome β5-GFP via the overexpression or knockdown of Yap. Scale bar, 10 μm. (c) HepG2 cells overexpressing or knockdown Yap were treated with 1 μg ml−1TM for 8 h and ER sizes were measured using an ER-tracker dye. Quantification of relative fluorescence intensity of ER-tracker dye of indicated cell samples was shown in the right panel. Data were assessed by Student’st-test and represented as mean±s.d.,n=3. *P<0.05, **P<0.01 compared with respective controls or as indicated. (d) TEMs of HepG2 cells transfected with Yap shRNA or scramble control shRNA followed by 1 μg ml−1TM treatment. The ‘N’ refers to nuclear and the arrow indicates the expanded ER compartment. ER thickness was quantified for the indicated TEM samples. Scale bar, 0.5 μm. Data were assessed by Student’st-test and represented as mean±s.d.n=24, ***P<0.001 compared with respective controls. (e) Intracellular Ca2+levels in HepG2 cells overexpressing or knockdown Yap were measured with flow cytometry using the Ca2+indicator Fluo-4 AM followed by 10 μM ionomycin treatment. Data are representative of at least three independent experiments. Figure 3: Yap regulates UPR signalling and ER size in a cell-intrinsic manner. ( a ) Western blot analysis of UPR and Hippo signalling elements of HepG2 cells overexpressing luciferase or Yap. ( b ) The assessment of the role of Yap in the morphological changes of the ER (GFP fluorescence) in response to 1 μg ml −1 TM treatment in HepG2 cells stably expressing cytochrome β5-GFP via the overexpression or knockdown of Yap. Scale bar, 10 μm. ( c ) HepG2 cells overexpressing or knockdown Yap were treated with 1 μg ml −1 TM for 8 h and ER sizes were measured using an ER-tracker dye. Quantification of relative fluorescence intensity of ER-tracker dye of indicated cell samples was shown in the right panel. Data were assessed by Student’s t -test and represented as mean±s.d., n =3. * P <0.05, ** P <0.01 compared with respective controls or as indicated. ( d ) TEMs of HepG2 cells transfected with Yap shRNA or scramble control shRNA followed by 1 μg ml −1 TM treatment. The ‘N’ refers to nuclear and the arrow indicates the expanded ER compartment. ER thickness was quantified for the indicated TEM samples. Scale bar, 0.5 μm. Data were assessed by Student’s t -test and represented as mean±s.d. n =24, *** P <0.001 compared with respective controls. ( e ) Intracellular Ca 2+ levels in HepG2 cells overexpressing or knockdown Yap were measured with flow cytometry using the Ca 2+ indicator Fluo-4 AM followed by 10 μM ionomycin treatment. 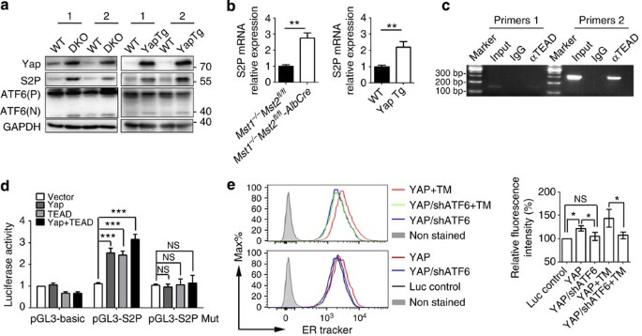Data are representative of at least three independent experiments. Figure 4: Yap regulates ER size through ATF6. Western blotting (a) or quantitative PCR (b) showing the expression levels of S2P, ATF6 (N) or total Yap in the livers ofMst1/2DKO andYaptransgenic mice. (c) Chromatin immunoprecipitation (ChIP) assay showing that TEAD bound to theS2Ppromoter in HepG2 cells. (d) Luciferase assay showing that Yap and/or TEAD enhanced WT but not TEAD binding sites-mutatedS2Ppromoter-driven luciferase activities. (e) HepG2 cells with or without the overexpression of Yap or knockdown of ATF6 were treated with 1 μg ml−1TM for 8 h and ER sizes were measured using an ER-tracker dye. Quantification of relative fluorescence intensity of ER-tracker dye of indicated cell samples was shown in the right panel. Data were assessed by Student’st-test and represented as mean±s.d.n=3. ns, not significant, *P<0.05, **P<0.01, ***P<0.001 compared with respective controls or as indicated. Data are representative of at least three independent experiments. Full size image Figure 4: Yap regulates ER size through ATF6. Western blotting ( a ) or quantitative PCR ( b ) showing the expression levels of S2P, ATF6 (N) or total Yap in the livers of Mst1/2 DKO and Yap transgenic mice. ( c ) Chromatin immunoprecipitation (ChIP) assay showing that TEAD bound to the S2P promoter in HepG2 cells. ( d ) Luciferase assay showing that Yap and/or TEAD enhanced WT but not TEAD binding sites-mutated S2P promoter-driven luciferase activities. ( e ) HepG2 cells with or without the overexpression of Yap or knockdown of ATF6 were treated with 1 μg ml −1 TM for 8 h and ER sizes were measured using an ER-tracker dye. Quantification of relative fluorescence intensity of ER-tracker dye of indicated cell samples was shown in the right panel. Data were assessed by Student’s t -test and represented as mean±s.d. n =3. ns, not significant, * P <0.05, ** P <0.01, *** P <0.001 compared with respective controls or as indicated. Data are representative of at least three independent experiments. Full size image Yap prevents ER stress-induced cell death and liver injury We next sought to assess the role of Yap in cell fate determination during ER stress. We found that the overexpression of Yap decreased, whereas its knockdown enhanced, cell apoptosis as induced by a 36-h, 2 μg ml −1 TM treatment ( Fig. 5a–d ). Following the TM treatment, the numbers of TUNEL (terminal deoxynucleotidyl transferase dUTP nick-end labelling)-positive cells and the indicators of liver tissue injury, such as serum alanine transaminase (ALT) and aspartate transaminase (AST) levels, were much lower in the Mst1/2 -deficient or Yap transgenic livers but were greatly increased in the Yap -deficient livers compared with those in the WT livers, indicating that Yap protects against TM-induced liver cell death and injury ( Fig. 5e–g ). Thus, Yap is required for cell survival during ER stress. Figure 5: Yap protects against ER stress-induced cell death and liver injury. Annexin V/DAPI staining and the cleavage of PARP in Yap knockdown ( a , b ) or overexpressing ( c , d ) HepG2 cells treated with 2 μg ml −1 TM for 36 h. Bar graphs show the quantifications of Annexin V-positive cells in indicated samples, n =3. ( e , f ) Haematoxylin and eosin (H&E) or TUNEL staining of liver tissue sections from the WT, Mst1/2 DKO, Yap Tg or Yap fl/fl -Alb-Cre knockout mice after a 3-day PBS or 0.5 mg kg −1 TM treatment ( e ). Scale bar, 20 μm. Bar graphs show the quantifications of TUNEL-positive cells in the livers, n =5 ( f ). ( g ). Bar graphs show the quantifications of the serum ALT and AST levels of WT, Mst1/2 DKO, Yap Tg or Yap fl/fl -Alb-Cre mice after 3-day PBS or 0.5 mg kg −1 TM treatment. Data were assessed by Student’s t -test and represented as mean±s.d. ns, not significant, * P <0.05, ** P <0.01, *** P <0.001 compared with respective controls or as indicated. Data are representative of at least three independent experiments. Full size image PERK-eIF2α-ATF4 axis regulates Yap transcription in UPR To determine the status of Hippo signalling in an acute UPR induction system, we treated HepG2 cells with 1 μg ml −1 TM for different lengths of time ( Fig. 6a ). Notably, a significant induction in Yap expression at the initial stage (before 12-h treatment) was observed after the TM treatment, but decreased expression occurred at the later stage (after 16-h treatment). In addition, phospho-Mob1, phospho-Lats1/2 and phospho-Yap levels gradually increased in response to prolonged ER stress induction, indicating that Hippo signalling was activated at the later stage of ER stress ( Fig. 6a and Supplementary Fig. 6a ). Similar findings were observed in HepG2 cells treated with thapsigargin, which is another ER stress inducer that depletes intracellular Ca 2+ stores ( Supplementary Fig. 6b ). 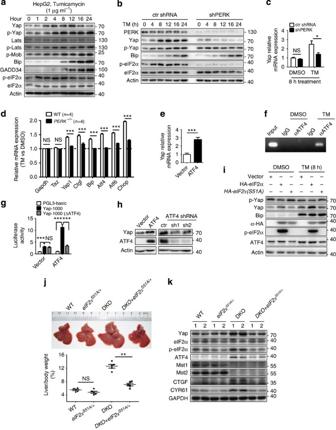Figure 6: PERK-eIF2α-ATF4 axis regulates Yap transcription during the UPR. (a) Western blot analysis of Hippo signalling elements in HepG2 cells treated with 1 μg ml−1TM for different lengths of time. Western blotting (b) or quantitative PCR (qPCR) (c) analysis of Yap expression in PERK-knockdown HepG2 cells treated with 1 μg ml−1TM for 8 h. (d) Extracted data from a previously reported microarray analysis52of UPR elements, Yap and CTGF levels in the livers of WT andPerkfl/fl-AlbCre(Perk−/−) mice followed by a 6-h 1 mg kg−1TM treatment. (e) qPCR analysis of Yap expression in HepG2 cells overexpressing ATF4. (f) Chromatin immunoprecipitation (ChIP) assay showing that ATF4 bound to theYappromoter in HepG2 cells followed by an 8-h 1 μg ml−1TM treatment. (g) Luciferase assay showing that ATF4 enhancedYap-1000-WT but notYap-1000-ΔATF4 promoter activity levels. (h) Western blotting showing that ATF4 regulated Yap expression. (i) Western blotting showing that eIF2α but not a mutated eIF2α (S51A) increased Yap protein levels in HepG2 cells. Knock-in of theeIF2α(S51A)gene led to significantly reduced liver masses and liver/body weight ratios in theMst1/2-deficient (DKO) mice (j) and decreased the protein levels of ATF4 and Yap in DKO livers (k),n=5. Data were assessed by Student’st-test and represented as mean±s.d. ns, not significant, *P<0.05, **P<0.01, ***P<0.001 compared with respective controls or as indicated. Data are representative of at least three independent experiments. Figure 6: PERK-eIF2α-ATF4 axis regulates Yap transcription during the UPR. ( a ) Western blot analysis of Hippo signalling elements in HepG2 cells treated with 1 μg ml −1 TM for different lengths of time. Western blotting ( b ) or quantitative PCR (qPCR) ( c ) analysis of Yap expression in PERK-knockdown HepG2 cells treated with 1 μg ml −1 TM for 8 h. ( d ) Extracted data from a previously reported microarray analysis [52] of UPR elements, Yap and CTGF levels in the livers of WT and Perk fl/fl -AlbCre ( Perk −/− ) mice followed by a 6-h 1 mg kg −1 TM treatment. ( e ) qPCR analysis of Yap expression in HepG2 cells overexpressing ATF4. ( f ) Chromatin immunoprecipitation (ChIP) assay showing that ATF4 bound to the Yap promoter in HepG2 cells followed by an 8-h 1 μg ml −1 TM treatment. ( g ) Luciferase assay showing that ATF4 enhanced Yap -1000-WT but not Yap -1000-ΔATF4 promoter activity levels. ( h ) Western blotting showing that ATF4 regulated Yap expression. ( i ) Western blotting showing that eIF2α but not a mutated eIF2α (S51A) increased Yap protein levels in HepG2 cells. Knock-in of the eIF2 α (S51A) gene led to significantly reduced liver masses and liver/body weight ratios in the Mst1/2 -deficient (DKO) mice ( j ) and decreased the protein levels of ATF4 and Yap in DKO livers ( k ), n =5. Data were assessed by Student’s t -test and represented as mean±s.d. ns, not significant, * P <0.05, ** P <0.01, *** P <0.001 compared with respective controls or as indicated. Data are representative of at least three independent experiments. Full size image PERK is required for the full induction of the UPR transcriptome in response to ER stress [5] . We found that the knockdown of PERK, but not ATF6 or IRE1α, significantly reduced Yap induction during ER stress ( Fig. 6b,c and Supplementary Fig. 6c,d ). We extracted a data set from a previously reported microarray characterization of livers from WT or liver-specific PERK knockout ( Perk −/− ) mice treated with or without TM [52] , and found that in addition to UPR elements such as ATF4, ATF6, Bip and CHOP, the mRNA levels of Yap and its target CTGF were also significantly upregulated in the TM-treated WT livers but not in the TM-treated Perk −/− livers ( Fig. 6d ). PERK-mediated eIF2α phosphorylation attenuates general protein synthesis but preferentially induces the translation of some key factors to promote the integrated stress response, including the transcriptional factor ATF4 (ref. 53 ). Interestingly, overexpression of ATF4 enhanced the transcriptional level of Yap ( Fig. 6e ), and the chromatin immunoprecipitation assay using the ATF4 antibody revealed that ATF4 could specifically bind to the Yap promoter in HepG2 cells following TM treatment ( Fig. 6f ). An analysis of the Yap promoter showed that one ATF4 binding site was present within its 1,000-bp promoter region (Yap-1,000) ( Supplementary Fig. 6f ). As expected, ATF4 overexpression significantly enhanced Yap promoter-driven luciferase activity and Yap protein levels, whereas the knockdown of ATF4 or the deletion of the ATF4 binding site decreased Yap expression or Yap -1,000 promoter-driven luciferase activity ( Fig. 6g,h ). The overexpression of eIF2α alone, but not non-phosphorylatable eIF2α (S51A), increased endogenous Yap protein levels with or without TM treatment ( Fig. 6i ). These data indicate that phosphorylated eIF2α plays a prominent role in the regulation of Yap expression under ER stress conditions. Importantly, the liver masses and the liver-to-body weight ratios significantly decreased in the DKO mice carrying the eIF2 α (S51A) knock-in mutation of only one allele ( Fig. 6j ) or the DKO mice infected with adenoviruses expressing eIF2α (S51A) (Ad-eIF2α (S51A)) compared with those of the green fluorescent protein (GFP)-expressing recombinant adenovirus (Ad-GFP)-treated animals ( Supplementary Fig. 7a ). Western blottings further confirmed that phospho-eIF2α-mediated signalling is required for Yap activation and liver growth ( Fig. 6k and Supplementary Fig. 7b–d ). Hippo signalling stabilises GADD34 and CreP proteins GADD34 expression is induced on prolonged ER stress induction ( Fig. 6a ) and it has been shown that GADD34 and its structural homologue, CReP, both associate with PP1 and facilitate the dephosphorylation of eIF2α, resulting in a negative feedback loop to recover protein synthesis during the ER stress [9] . The expression levels of GADD34 and CReP dramatically decreased in the DKO livers compared with those in the WT livers ( Fig. 7a and Supplementary Fig. 8a ). Overexpressed Mst2 in HepG2 cells resulted in increased levels of total GADD34 and CReP, and a dramatic reduction in eIF2α phosphorylation ( Fig. 7b and Supplementary Fig. 8b ). We performed co-immunoprecipitation assays to determine whether the Flag-tagged components of the Hippo pathway, including TAZ, Yap, Lats1, Mst2, Mob1a, Rassf1a and WW45, could bind specifically to haemagglutinin (HA)-tagged GADD34, and found that only Flag-Lats1 was associated with HA-GADD34 ( Supplementary Fig. 8c ). A substantial increase in phospho-eIF2α and decrease in GADD34 and CReP levels were observed in Lats1/2-deficient mouse embryonic fibroblasts. Conversely, the overexpression of Lats1 in HepG2 cells significantly decreased phospho-eIF2α and increased GADD34 and CReP levels ( Fig. 7c and Supplementary Fig. 8d ). A previous study suggested that the transient nature of GADD34, which is rapidly polyubiquitinated and degraded by the 26S proteasome, plays an important role in determining cell survival/cell death decisions [54] . Our study showed that Lats1 did not regulate the mRNA levels of GADD34 and CReP but did regulate the stabilities of the GADD34 and CReP proteins, because the overexpression of Lats1 resulted in a substantial reduction in GADD34 and CReP ubiquitination ( Fig. 7d and Supplementary Fig. 8e,f ). 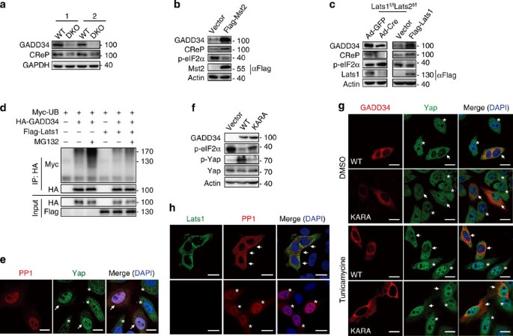Figure 7: GADD34 stabilized by Hippo signalling results in increased Yap phosphorylation and cytoplasmic retention. Western blotting showing the dramatic reduction of GADD34/CReP in theMst1/2-deficient livers (a) or in the Lats1/2-null mouse embryonic fibroblasts (c). The overexpression of Mst2 (b) or Lats1 (c) resulted in increased GADD34/CReP and decreased phospho-eIF2α levels in HepG2 cells. (d) Western blotting showing that overexpression of Lats1 decreased GADD34 ubiquitination in HepG2 cells. (e) Overexpression of PP1 promoted Yap nuclear translocation. The subcellular localization of transfected PP1 (red) and endogenous Yap (green) was determined by immunofluorescence staining along with DAPI for DNA (blue) in HepG2 cells. Cell transfected with or without PP1 was indicated with arrow or star, respectively. Scale bar, 10 μm. (f) Western blotting showing that GADD34 (WT) but not GADD34 (KARA) downregulated phospho-eIF2α and increased phospho-Yap levels in HepG2 cells. (g) Immunofluorescence staining showing that GADD34 (WT, red) but not GADD34 (KARA, red) promoted endogenous Yap (green) cytoplasmic retention in HepG2 cells treated with 1 μg ml−1TM for 8 h. Cells transfected with GADD34 (WT or KARA) and control cells were indicated with arrow and star, respectively. Scale bar, 10 μm. (h) The overexpression of Lats1 resulted in the cytoplasmic retention of PP1 in HepG2 cells. The subcellular localization of transfected PP1 (red) was determined in HepG2 cells with or without Lats1 overexpression by immunofluorescence staining along with DAPI for DNA (blue). Cell transfected with or without Lats1 was indicated with arrow or star, respectively. Scale bar, 10 μm. Data are representative of at least three independent experiments. Figure 7: GADD34 stabilized by Hippo signalling results in increased Yap phosphorylation and cytoplasmic retention. Western blotting showing the dramatic reduction of GADD34/CReP in the Mst1/2 -deficient livers ( a ) or in the Lats1/2-null mouse embryonic fibroblasts ( c ). The overexpression of Mst2 ( b ) or Lats1 ( c ) resulted in increased GADD34/CReP and decreased phospho-eIF2α levels in HepG2 cells. ( d ) Western blotting showing that overexpression of Lats1 decreased GADD34 ubiquitination in HepG2 cells. ( e ) Overexpression of PP1 promoted Yap nuclear translocation. The subcellular localization of transfected PP1 (red) and endogenous Yap (green) was determined by immunofluorescence staining along with DAPI for DNA (blue) in HepG2 cells. Cell transfected with or without PP1 was indicated with arrow or star, respectively. Scale bar, 10 μm. ( f ) Western blotting showing that GADD34 (WT) but not GADD34 (KARA) downregulated phospho-eIF2α and increased phospho-Yap levels in HepG2 cells. ( g ) Immunofluorescence staining showing that GADD34 (WT, red) but not GADD34 (KARA, red) promoted endogenous Yap (green) cytoplasmic retention in HepG2 cells treated with 1 μg ml −1 TM for 8 h. Cells transfected with GADD34 (WT or KARA) and control cells were indicated with arrow and star, respectively. Scale bar, 10 μm. ( h ) The overexpression of Lats1 resulted in the cytoplasmic retention of PP1 in HepG2 cells. The subcellular localization of transfected PP1 (red) was determined in HepG2 cells with or without Lats1 overexpression by immunofluorescence staining along with DAPI for DNA (blue). Cell transfected with or without Lats1 was indicated with arrow or star, respectively. Scale bar, 10 μm. Data are representative of at least three independent experiments. Full size image GADD34 regulates Yap activity via modulating PP1 location GADD34 is present in the cytoplasm and several membrane compartments, including the ER, mitochondria and Golgi bodies [55] . In association with PP1, GADD34 regulates the PERK pathway via the dephosphorylation of eIF2α. We observed that PP1 was exclusively localized to the nucleus and promoted Yap nuclear translocation in HepG2 cells ( Fig. 7e and Supplementary Fig. 9a ), and GADD34 was induced at the later stage of ER stress, which correlated with increased phosphor-Yap levels ( Fig. 6a ). To explore the effects of the GADD34/PP1 complex on the regulation of Yap phosphorylation, we transfected HepG2 cells with the WT form or the KARA form of GADD34, which fails to interact with PP1 due to a mutation in the highly conserved KVRF PP1-binding sequence [56] . Surprisingly, the WT GADD34 promoted eIF2α dephosphorylation but enhanced Yap phosphorylation, whereas the KARA form did not affect phospho-Yap levels ( Fig. 7f ). Immunofluorescence staining confirmed that the WT GADD34 blocked Yap nuclear translocation following the TM treatment, while the KARA form did not ( Fig. 7g and Supplementary Fig. 9b ). Further analyses revealed that PP1 was largely excluded from the nuclear compartment in the WT GADD34-transfected cells, but was mainly distributed in the nuclei of the cells transfected with the KARA form of GADD34 ( Supplementary Fig. 9c ). HepG2 cells overexpressing Last1 or Mst2 exhibited increased levels of GADD34 and reduced nuclear PP1 levels ( Fig. 7h and Supplementary Fig. 9d,e ). These results suggest that Yap dephosphorylation by PP1 may occur in the nuclear compartment, and that GADD34 blocks PP1 nuclear translocation. Following the TM treatment, the increased GADD34 levels correlated with the gradually enhanced phospho-Yap levels, which were not observed in the GADD34-knockdown cells ( Fig. 8a and Supplementary Fig. 9f ). The knockout of GADD34 consistently promoted Yap expression, decreased phospho-Yap and reduced UPR-induced cell death ( Fig. 8b,c and Supplementary Fig. 9g ). Conversely, overexpression of GADD34 in HepG2 cells exhibited increased apoptotic events, which are rescued by coexpression of Yap(S127A) activated form ( Supplementary Fig. 9h ). Furthermore, the DKO mice infected with adenoviruses expressing GADD34 (Ad-GADD34) but not Ad-GFP exhibited enhanced levels of phospho-Yap in their livers, dramatically reduced liver masses and decreased the liver-to-body weight ratios ( Fig. 8d–f ). 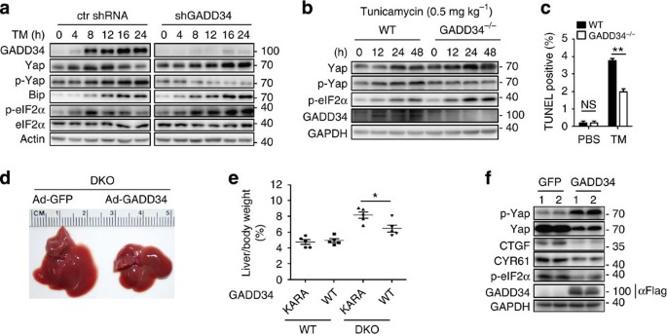Figure 8: GADD34 regulates Yap activity and liver size. Western blotting showing that the knockdown of GADD34 in HepG2 cells treated with 1 μg ml−1TM for indicated times (a) or the knockout of GADD34 in the livers followed by 0.5 mg kg−1TM treatment (b) reduced phospho-Yap and increased Yap levels. (c) Bar graphs show the quantifications of TUNEL-positive cells in the GADD34 knockout and WT control livers. (d–f) The liver masses of theMst1/2DKO mice infected with adenoviruses expressing GADD34 (Ad-GADD34) or control GFP (Ad-GFP) (d). The liver/body weight ratios of the WT orMst1/2DKO mice infected with the indicated adenoviruses were quantified as shown,n=5 (e). Decreased phospho-eIF2α and increased phospho-Yap levels were confirmed in the Ad-GADD34-treated livers (f). Data are representative of at least three independent experiments. Data were assessed by Student’st-test and represented as mean±s.d.. ns, not significant, *P<0.05, **P<0.01, compared with respective controls or as indicated. Figure 8: GADD34 regulates Yap activity and liver size. Western blotting showing that the knockdown of GADD34 in HepG2 cells treated with 1 μg ml −1 TM for indicated times ( a ) or the knockout of GADD34 in the livers followed by 0.5 mg kg −1 TM treatment ( b ) reduced phospho-Yap and increased Yap levels. ( c ) Bar graphs show the quantifications of TUNEL-positive cells in the GADD34 knockout and WT control livers. ( d – f ) The liver masses of the Mst1/2 DKO mice infected with adenoviruses expressing GADD34 (Ad-GADD34) or control GFP (Ad-GFP) ( d ). The liver/body weight ratios of the WT or Mst1/2 DKO mice infected with the indicated adenoviruses were quantified as shown, n =5 ( e ). Decreased phospho-eIF2α and increased phospho-Yap levels were confirmed in the Ad-GADD34-treated livers ( f ). Data are representative of at least three independent experiments. Data were assessed by Student’s t -test and represented as mean±s.d.. ns, not significant, * P <0.05, ** P <0.01, compared with respective controls or as indicated. Full size image Taken together, our data suggest that GADD34 may serve as a docking platform for PP1, which preferentially dephosphorylates eIF2α in the cytoplasm, and that it may block PP1-mediated Yap dephosphorylation in the nuclear compartment. Thus, during the ER stress, Hippo signalling stabilizes GADD34 to inhibit the activation of Yap. PERK-eIF2α-Yap signalling is implicated in HCC development ER homeostasis is dysregulated in a variety of cancers. Enhanced UPR signalling was observed in the DKO livers, which eventually developed HCC. To mimic the effects of chronic ER stress, we treated HepG2 cells with a low dose of TM (10 ng ml −1 ) for 5 passages for up to 15 days. Compared with the untreated samples, the low-dose TM-treated HepG2 cells exhibited consistently increased total Yap levels but gradually decreasing phospho-Yap and phospho-Mob1 levels, which are downstream substrates of the Mst1/2 kinases, indicating that Hippo signalling is inhibited in cells undergoing chronic ER stress ( Fig. 9a and Supplementary Fig. 10a ). HepG2 cells undergoing chronic ER stress that was induced by the low-dose TM treatment grew more vigorously and formed larger tumour masses in the nude mice compared with the dimethylsulfoxide-treated control cells ( Fig. 9b,c ). In addition, the knockdown of Yap promoted cell death under chronic ER stress ( Supplementary Fig. 10b ). These results indicate that Yap is required for cell growth and survival under chronic ER stress. 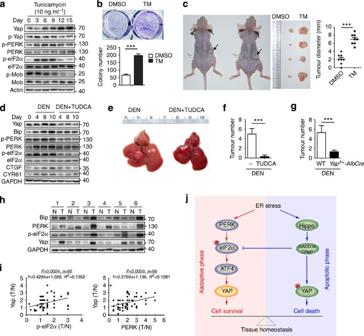Figure 9: Elevated PERK-eIF2α-Yap signalling is associated with the development of mouse and human HCC. (a–c) A low dose of TM promotes cell hyperproliferation. Western blot analysis of PERK signalling and Yap levels in HepG2 cells treated with a low dose of TM (10 ng ml−1) for the indicated number of days (a). Low-dose TM-treated HepG2 cells exhibited the formation of significantly more colonies (b) and formed tumours of larger masses in the nude mice (c) compared with the dimethylsulfoxide (DMSO)-treated control cells,n=8. The black arrow indicates the TM-treated tumour cells; the white arrow denotes the control cells. Data were assessed by Student’sttest and represented as mean±s.d. ***P<0.001. (d) Western blotting with the indicated antibodies in liver tissues isolated from DEN- or DEN-plus-TUDCA-treated mice. (e,f) TUDCA treatment reduced liver masses (e) and the numbers of HCC tumors (f) in DEN-challenged mice,n=8. Data assessment is same as inc. ***P<0.001. (g)Yapfl/+-AblCremice exhibited significantly reduced numbers of DEN-induced HCC tumours compared with control WT mice. Data assessment is same as inc. ***P<0.001. (h,i) Western blot analysis of Bip, PERK, phospo-eIF2α and Yap in liver cancer tissue (T) and non-tumorous liver tissue (N) isolated from one patient. A total of six representative paired samples are shown (h). SeeSupplementary Fig. 11for the remaining 60 paired samples. The intensities of the immunoblot bands were quantified using the Imagine gel software. The ratio of the relative expression of the indicated proteins in the T and N from one patient was plotted and applied with the linear regressiont-test (i). (j) A proposed working model for the interplay of the Hippo pathway and the UPR signalling for cell fate determination. Under ER stress conditions, the PERK-mediated eIF2α phosphorylation increases ATF4 expression for the subsequent induction of Yap. Activated Yap increases UPR activity, the size and Ca2+storage capacity of ER for cell survival. When ER stress is excessive and homeostasis is not restored, Hippo signalling is activated for stabilizing GADD34/CReP proteins, which assemble with PP1 to form a complex to dephosphorylate eIF2α and reduces the PP1 abundance in the nucleus. In the end, increased Yap phosphorylation inhibits UPR activity and ER membrane expansion and eventually promotes cell death. Figure 9: Elevated PERK-eIF2α-Yap signalling is associated with the development of mouse and human HCC. ( a – c ) A low dose of TM promotes cell hyperproliferation. Western blot analysis of PERK signalling and Yap levels in HepG2 cells treated with a low dose of TM (10 ng ml −1 ) for the indicated number of days ( a ). Low-dose TM-treated HepG2 cells exhibited the formation of significantly more colonies ( b ) and formed tumours of larger masses in the nude mice ( c ) compared with the dimethylsulfoxide (DMSO)-treated control cells, n =8. The black arrow indicates the TM-treated tumour cells; the white arrow denotes the control cells. Data were assessed by Student’s t test and represented as mean±s.d. *** P <0.001. ( d ) Western blotting with the indicated antibodies in liver tissues isolated from DEN- or DEN-plus-TUDCA-treated mice. ( e , f ) TUDCA treatment reduced liver masses ( e ) and the numbers of HCC tumors ( f ) in DEN-challenged mice, n =8. Data assessment is same as in c . *** P <0.001. ( g ) Yap fl/+ -AblCre mice exhibited significantly reduced numbers of DEN-induced HCC tumours compared with control WT mice. Data assessment is same as in c . *** P <0.001. ( h , i ) Western blot analysis of Bip, PERK, phospo-eIF2α and Yap in liver cancer tissue (T) and non-tumorous liver tissue (N) isolated from one patient. A total of six representative paired samples are shown ( h ). See Supplementary Fig. 11 for the remaining 60 paired samples. The intensities of the immunoblot bands were quantified using the Imagine gel software. The ratio of the relative expression of the indicated proteins in the T and N from one patient was plotted and applied with the linear regression t -test ( i ). ( j ) A proposed working model for the interplay of the Hippo pathway and the UPR signalling for cell fate determination. Under ER stress conditions, the PERK-mediated eIF2α phosphorylation increases ATF4 expression for the subsequent induction of Yap. Activated Yap increases UPR activity, the size and Ca 2+ storage capacity of ER for cell survival. When ER stress is excessive and homeostasis is not restored, Hippo signalling is activated for stabilizing GADD34/CReP proteins, which assemble with PP1 to form a complex to dephosphorylate eIF2α and reduces the PP1 abundance in the nucleus. In the end, increased Yap phosphorylation inhibits UPR activity and ER membrane expansion and eventually promotes cell death. Full size image Diethylnitrosamine (DEN), which is a hepatic procarcinogen, is frequently used to induce HCC in mice. Consistent with our observations in the DKO animals, the expression levels of Yap, Bip, phospho-PERK and phospho-eIF2α were also highly upregulated in the DEN-treated livers compared with the control livers ( Fig. 9d and Supplementary Fig. 10c ). To study the effects of TUDCA on DEN-induced HCC, WT mice were treated with PBS or TUDCA twice per week following the DEN injection. We found that the expression levels of Yap, CTGF, CYR61, phospho-PERK and phospho-eIF2α in the DEN-treated livers were substantially downregulated following the TUDCA treatment ( Fig. 9d and Supplementary Fig. 10d ). This treatment significantly decreased the liver masses and the numbers of HCC tumours in the DEN-challenged mice ( Fig. 9e,f ). In addition, the deletion of one Yap allele in the mice livers significantly reduced the number of DEN-induced HCC tumours ( Fig. 9g ). These results indicate that UPR signalling and Yap play an important role in DEN-induced HCC development. We have previously shown that Hippo signalling is commonly lost in human HCCs in association with increased Yap expression and reduced phospho-Yap levels [23] . Our current study demonstrates that sustained ER stress responses correlate with the expression and activation of Yap in human HCC samples. We examined 66 pairs of liver-derived tumorous (T) and adjacent non-tumorous (N) tissues. Higher T-to-N ratios of PERK, phospho-eIF2α and Yap expression were associated with HCC development ( Fig. 9h and Supplementary Fig. 11a,b ). The T-to-N ratio of Yap expression was significantly correlated with those of PERK and eIF2α ( Fig. 9i ). These results suggest that methods such as the TUDCA treatment, which lead to the increased expression of Yap in human HCC, probably due to elevated PERK signalling and thus the attenuation of UPR signalling, are promising therapeutic strategies for the treatment of human HCC. Activation of the UPR by ER stress reduces the unfolded protein load in the ER through several pro-survival mechanisms. When ER stress is excessive and homeostasis is not restored, the UPR triggers apoptosis to eliminate the damaged cells and the failure of cell death may lead to oncogenesis [2] . In this study, we uncovered a physiological role of Yap in maintaining ER homeostasis and demonstrated that the synergistic effects of Hippo signalling and PERK branch of the UPR are critical for cell fate determination during ER stress, in which the induction and activation of Yap is the key event ( Fig. 9j ). The liver is one of the major secretory organs in the body. Its functions include regulation of glucose homeostasis, lipid metabolism and drug detoxification. The UPR is indispensable and actively involved in hepatocyte activities, ensuring their proper functioning and survival [57] . We found that Mst1/2 - or WW45 -deficient livers exhibited greatly enhanced UPRs, resulting in gradually increased levels of Yap expression that depended on the induction of PERK signalling, which is required for cell survival [58] . The canonical UPR led to the PERK-dependent phosphorylation of eIF2α at S51, which suppresses general protein synthesis but selectively promotes the translation of ATF4, to alleviate ER stress. A previous study showed that ER stress-induced apoptosis is enhanced in Perk −/− and eIF2 α (S51A) mutant cells through poorly understood mechanisms [58] . Our present work shows that Yap could be a major factor that acts downstream of PERK-eIF2α-ATF4 signalling for cell survival. In addition to enhance ATF6 signals, we found that ATF4 promotes Yap transcriptional induction in cells experiencing ER stress, and activated Yap further promotes the cleavage and activation of ATF6 for ER biogenesis. Cells treated with ER stress inducers exhibited initially decreased but then increased phospho-Yap levels, and these changes correlate with the adaptive and apoptotic phases of the UPR. We discovered that PP1, which can act as a phosphatase for either eIF2α or Yap, is a key molecular switch that regulates the phosphorylation status of Yap. PP1 is typically localized to the nucleus, where it is available to dephosphorylate Yap and promote its activation for cell survival during the early stage of the UPR. Prolonged ER stress leads to sustained PERK signalling, which induces the expression of GADD34. GADD34 then forms a complex with PP1 in the outer layer of the ER membrane to dephosphorylate eIF2α, thus participating in a negative feedback loop to reduce Yap expression and activation. In addition to directly phosphorylating Yap at Ser127, Hippo signalling stabilizes GADD34 and increases the assembly of the ER-associated GADD34/PP1 complex to reduce the abundance of PP1 in the nucleus, thus resulting in increased phospho-Yap and eventually triggering cell apoptosis. Thus, our present findings demonstrate that the expression and activation of Yap is modulated through several novel mechanisms. Yap may act as a switch between the pro-survival and pro-apoptotic responses of the UPR response. Recent studies have shown that Yap can promote cell death by binding p73 to activate PML transcription [59] , [60] . Moreover, we previously reported that Hippo signalling decreases Yap expression to promote cell apoptosis by inhibiting GABP transcriptional activity [42] . Thus, the evaluation of the potential role of these Yap regulators in cell fate determination during ER stress is of interest. Individual UPR pathways have been linked to cancers arising from diverse tissues [61] , [62] . We observed that the expression levels of PERK and, subsequently, phospho-eIF2α were positively correlated with increased Yap expression levels in most human HCC tumour samples. In addition to PERK signalling, the ATF6 branch of the UPR, including full-length and cleaved ATF6, was also greatly upregulated in the Mst1/2-deficient livers. ATF6 is transported from the ER to the Golgi apparatus, where it is processed by regulated intramembrane proteases to release a cleaved cytosolic fragment (ATF6(N)) that regulates the transcriptional expression of ER chaperones and XBP1 to promote cell survival [63] . A recent report showed that the PERK-eIF2α-ATF4 pathway is required for activation of ATF6 and it’s target genes through facilitating the synthesis of ATF6 and it’s trafficking from the ER to the Golgi [52] . Thus, the increased ATF6 signals that were detected in the Mst1/2-deficient livers may have simply been due to enhanced PERK signalling resulting from the inactivation of Hippo signalling. Yap can further promote the cleavage and activation of ATF6 by enhancing the expression of S2P. The activation of ATF6 plays a role in triggering Xbp1-independent ER expansion [51] . In the current study, the activation of Yap resulting from the deletion of Mst1/2 in the mouse livers or its overexpression in HepG2 cells resulted in greatly increased ER sizes, which may have been due to the activation of ATF6 in these tissues or cells. It is interesting to note that the activation of the IRE1α branch of UPR was greatly blocked in the Mst1/2 -deficient livers, in which tumours eventually developed, although previous studies indicated that Xbp1, the downstream effector of IRE1α signalling, is required for ER membrane expansion and play pro-survival role [64] , [65] , [66] . A recent study showed that IRE1α-Xbp1 signalling is turned off following prolonged ER stress, whereas PERK signalling can be sustained [67] . More recently, hyperactivation of IRE1α branch was shown to cause cell death [68] . Thus, we speculate that the IRE1α activity is reduced to prevent cell apoptosis in Mst1/2 knockout liver. Given that Xbp1 expression is increased due to the activation of PERK-ATF6 axis in Mst1/2-deficient liver and Xbp1 is also important for expansion of the ER compartment, the role of Xbp1 in Mst1/2 mutant-driven liver cell malignant transformation need to be determined in the future study. Our observations suggest the presence of continued and perpetual ER stress in the liver, in the absence of Hippo signalling. Interestingly, treatment with the BA TUDCA, which is a chemical chaperone that alleviates ER stress, abolished the HCC formation that was induced by the carcinogenic (DEN) or genetic ( Mst1/2 knockout) approaches. Thus, our study has provided direct and robust evidence showing that ER stress may be mitogenic and oncogenic, at least in the absence of Hippo signalling. TUDCA treatment could be a potential therapeutic strategy for the treatment of human HCC. Animals The Mst1 , Mst2 , WW45 and Yap gene conditional knockout and the Yap (S127A) transgenic mice were previously described [23] , [25] , [31] . WT C57BL/6, albumin (Alb)-Cre mice (stock number 003574) and eIF2α (S51A) knock-in mice (stock number 017601) [69] were originally purchased from The Jackson Laboratory. All mice were maintained under specific pathogen-free conditions at the Xiamen University Laboratory Animal Center. This mouse experiment was approved by the Institutional Animal Care and Use Committee and was in strict accordance with good animal practice, as defined by the Xiamen University Laboratory Animal Center. Generation of GADD34 knockout mice by TALEN TALEN (transcription activator-like effector nuclease) constructs were linearized at the PVU2 site. In vitro transcripts were generated using the T7 Message Max Kit and Poly(A) Tailing Kit (Epicentre, IL, USA) following the manufacturer’s instructions. Washed and dried RNA was dissolved in water and the concentration was determined using a spectrophotometer. TALEN mRNA was injected into fertilized mouse eggs at a concentration of 4 ng μl −1 . The injected eggs were then transferred to pseudopregnant females at 0.5 days post coitum. DNA samples from the tails of the newborn mice were amplified with PrimeSTAR DNA Polymerase (Takara, Dalian, China) and the PCR products were sequenced for the screening of heterozygous or knockout descendants. Chemicals The TM, thapsigargin and dithiothreitol were obtained from Sigma-Aldrich (St Louis, MO, USA). The TUDCA was purchased from EMD Millipore (Billerica, MA, USA). Cell culturing The HepG2 and 293T cell lines were obtained from ATCC and cultured in DMEM (Invitrogen, Carlsbad, CA, USA) supplemented with 10% fetal bovine serum and 1 × penicillin/streptomycin. Human liver and HCC samples Human samples were obtained with informed consent from the human tissue banks of the Xiamen Hospital of Traditional Chinese Medicine and Zhongshan Hospital of Xiamen University. All experiments were performed with the approval of the Xiamen University Review Board. Snap-frozen biopsies from specimens of normal liver tissue (distant from the tumour) and HCC were collected. The diagnosis of HCC or normal liver was confirmed based on histological findings by independent pathologists. Isolation and culture of mouse hepatocytes Mouse primary hepatocytes were isolated by the two-step liver perfusion method. Briefly, the mouse was anaesthetized with intraperitoneal injection of xylazine (10 mg kg −1 body weight) and ketamine (100 mg kg −1 body weight). The abdomen was then cut open and the portal vein was catheterized. The liver was first perfused in situ with D-Hank’s buffered solution (containing 0.5 mM EGTA, pre-warmed to 37 °C) for 8–10 min with the inferior vena cava cut for drainage and then perfused for 5 min with 0.12 PZ-U ml −1 collagenase perfusate (containing 2 mM Ca 2+ ). The livers were extirpated and transferred into plates filled with DMEM at 4 °C. The hepatic capsules were torn and the livers were gently shaken to help the cells detach. The cell suspension was collected and filtered through 70-μm cell strainers (BD Falcon, Bedford, USA). Cell viability, as determined by trypan blue exclusion, was generally >90%. The cells were plated in 24-well gelatin-coated plates (8 × 10 4 ) in Williams’ Medium E (Invitrogen) containing 10% fetal bovine serum, 100 U ml −1 penicillin/streptomycin and 1 × 10 −7 M insulin, and cultured at 37 °C with 5% CO 2 . ER stress induced in cells and animals HepG2 cells were treated with TM as indicated in the results. ER stress was induced in mice by a single intraperitoneal (IP) injection with TM at 0.5 mg per kg body weight. Control mice were treated by injection with an equal volume of PBS. Three days post injection, all mice were anaesthetized and killed by decapitation and serum was collected from mice via cardiac puncture. Liver samples were either immersion fixed overnight in 4% paraformaldehyde in PBS (pH 7.3) for subsequent histological analysis or were snap frozen in liquid nitrogen for subsequent biochemical analyses. ALT and AST levels were determined in blood specimens with the use of an ALT/AST assay kit (20030106; NJJCBio, Beijing, China). Administration of TUDCA in mice To determine the effect of TUDCA on liver size control, 8-week-old WT or Mst1/2 DKO mice were treated with 100 mg kg −1 TUDCA (EMD Millipore) by IP injection once a day for 2 weeks. To determine the effect of TUDCA on the development of liver cancer in the Mst1/2 DKO mice, 8-week-old mice were treated with 250 mg kg −1 TUDCA by IP injection twice a week for 10 weeks. Control mice received the same volume of PBS by IP injection at same time points. Liver tissues used for RNA purification, protein extraction or histology were harvested at the indicated times. mRNA sequencing The mRNA-Seq experiments were performed by Novogene (Beijing, China). mRNA-seq library is prepared for sequencing using standard Illumina protocols. Briefly, total RNAs from primary mouse hepatocytes with or without 100 μM TUDCA treatment are isolated using TRIzol reagent (Invitrogen) and treated with RNase-free DNase I (New England Biolabs, MA, USA), to remove any contaminating genomic DNA. mRNA extraction is performed using Dynabeads oligo(dT) (Invitrogen Dynal). Double-stranded complementary DNAs are synthesized using Superscript II reverse transcriptase (Invitrogen) and random hexamer primers. The cDNAs are then fragmented by nebulization and the standard Illumina protocol is followed thereafter, to create the mRNA-seq library. For the data analysis, basecalls are performed using CASAVA. Reads are aligned to the genome using the split read aligner TopHat (v2.0.7) and Bowtie2, using default parameters. HTSeq is used for estimating their abundances. TEM and quantification for ER thickness The mouse liver mass was sliced to small pieces and fixed in a PBS solution with 2.5% glutaraldehyde (v/v) immediately on ice for 2 h. The primarily fixed samples were further sliced to a volume no larger than 2 mm 3 , rinsed with PBS for three times and then kept in 1% osmium tetraoxide (v/v) for 1 h for secondary fixation. After dehydration in a series of concentrations of ethanol, the tissues were finaly embedded in Embed 812 resin. Thin sections were cut on an ultramicrotome (LKB, Sweden), mounted on nickel grids, stained with saturated uranyl acetate and Reynolds lead citrate, and then examined with electron microscopy JEM2100HC (Jeol Ltd, Japan). For culture cells, HepG2 cells were treated as indicated, trypsinized, pelleted by centrifugation at 3,000 r.p.m. and then primarily fixed in a cold fixing solution containing 2.5% glutaraldehyde for 2 h. In addition, the following steps were exactly as that for liver samples. The ER thickness was quantified by measuring the distance between two membranes of the ER lumen in the TEM photographs. Briefly, values for the distance between the two membranes of ER lumen from randomly chosen five areas of each TEM photograph were averaged. The measurements from total 24 photographs (8 photographs per sample/mouse and 3 samples/mice per group) were displayed. Generation of recombinant adenovirus-encoded GADD34 or eIF2α S51A Recombinant adenovirus was generated as described previously [42] . Briefly, the GADD34 or eIF2α cDNA was subcloned into the multicloning site of the AdTrack-CMV shuttle vector, which contains a GFP as a reporter gene. The GADD34 or eIF2a cDNA was placed specifically between the KpnI and XhoI restriction sites between the cytomegalovirus promoter and polyadenylation sequences. The resultant plasmid was linearized by digestion with PmeI endonuclease and cotransformed into Escherichia coli BJ5183 cells with the AdEasy-1 adenoviral plasmid, which contains the entire genomic sequences of adenovirus serotype Ad5, except the nucleotides encompassing the E1 and E3 genes. Recombinant bacteria were selected by kanamycin resistance and the recombination was confirmed by a PacI endonuclease restriction analysis. The Ad-GFP was constructed similarly. Subsequently, the verified clone was amplified, linearized with PacI and transfected into HEK293A packaging cells. The recombinant adenovirus was released from the cells by four freeze–thaw–vortex cycles 14–20 days post transfection, amplified by further rounds of infection of HEK293A packaging cells and purified by CsCl ultracentrifugation. Stocks of purified adenovirus were titred by counting the number of plaque-forming units. The recombinant adenoviruses (2 × 10 9 pfu in 200 μl PBS) were injected into 6- to 8-week-old male mice via the tail vein. Transfection and luciferase reporter assays Cells cultured in 12-well plates were transfected with the indicated plasmids using Lipofectamine 2000 (Invitrogen). At 48 h post transfection, cells were washed with PBS and lysed in Reporter Lysis Buffer (Invitrogen). Luciferase reporter activities were measured in triplicate using the Dual-Luciferase reporter assay system (Promega, Madison, WI, USA), according to the manufacturer’s protocol, and quantified using the GloMax 96-well plate luminometer (Promega). The firefly luciferase to Renilla luciferase ratios were determined and defined as the relative luciferase activity. shRNA and lentiviral infection Short hairpin RNA (shRNA) plasmids against human PERK , ATF6 , IRE1 α, Gadd34 and Yap were purchased from Open Biosystems (Huntsville, AL, USA). Human TRIPZ lentiviral inducible shRNA plasmids V3LHS_639173(sh1), V3LHS_639175(sh2), V3LHS_639179(sh3), V3LHS_639180(sh4), V3LHS_645454(sh5) and V3LHS_645455(sh6) are specific for human PERK . The shRNA plasmids V3THS_370378 (sh1), V3THS_370379 (sh2), V3THS_370382 (sh3), V2THS_210688 (sh4) and V2THS_250549 (sh5) are specific for human Gadd34 . The best efficient shRNAs are PERK (sh1) and Gadd34 (sh1), respectively. The shRNA plasmids V3LHS_365124 (sh1), V3LHS_365119 (sh2) and V3THS_365120 (sh3) are specific for human ATF6 . The shRNA plasmids V2THS_19871 (sh1), V2THS_113771 (sh2), V2THS_311696 (sh3), V2THS_311698 (sh4) and V2THS_311699 (sh5) are specific for human IRE1 α. shRNA ATF6 (sh3) and shRNA ATF6 (sh3) are the best. Yap shRNA was described previously [23] . The TRIPZ lentiviral-inducible empty vector (pIN-10-RFP) was used as the control vector. Lentivirus was produced by co-transfecting 293T cells with the shRNA vector, VSV-G and Δ8.9 plasmids using Lipofectamine 2000 (Invitrogen). Viral supernatant was harvested at 48–72 h post transfection, passed through a 0.45-μm filter, diluted 2:3 with fresh medium containing 8 μg ml −1 polybrene and used to infect the target cells at 80% confluence. Selection with puromycin (2 μg ml −1 ) was initiated at 48 h after viral infection. The mRNA levels were quantified by quantitative RT–PCR and protein expression was visualized by immunoblotting. Real-time quantitative PCR One microgram of total RNA from the liver tissue or cells was reverse transcribed with oligo dT and Superscript III reverse transcriptase (Invitrogen). Real-time quantitative PCR was performed as described previously [23] , using a BioRad iQ SYBR Green Supermix kit and the BioRad iCycler iQ system (BioRad, Hercules, CA, USA). All runs were accompanied by the internal control Gapdh gene. The samples were run in triplicate and normalized to GAPDH using a ΔΔ cycle threshold-based algorithm, to provide arbitrary units representing relative expression levels. The primer sequences for specific genes are shown in Supplementary Table 2 . Each graph is representative of at least three independent experiments. Immunoblotting The proteins were separated by PAGE, transferred onto a polyvinylidene difluoride membrane and then identified by immunoblotting using the indicated primary antibodies with 1:1,000 dilutions or as indicated. Antibodies against phospho-Yap (S127) (4911), HA (3724), GFP (2555), GAPDH (2118), CHOP(2892), MBTPS2(2157), Bip(3177), IRE1α(3294), PERK(5683), phospho-PERK (Thr980) (3179), phospho-eIF2α (Ser51) (3597), eIF2α (9722), GCN2 (3302), phospho-PP1a (Thr320) (2581), PP1a(2582) and eIF2Bɛ (3595) were obtained from Cell Signaling (Beverly, MA, USA). Antibodies against CReP (14634-1-AP), GADD34 (10449-1-AP), ATF4 (60035-1-lg), eIF2AK1 (20499-1-AP) and eIF2AK2 (18244-1-AP) were obtained from Proteintech Group Inc. (Wuhan, China). The ATF6 (ab11909) and phospho-IRE1a (S724) (ab48187) antibodies were obtained from Abcam (Cambridge, MA, USA). Antibodies against CTGF (sc14939), XBP1 (M-186) (sc-7160) and phospho-PERK (Thr 981) (sc32577) were obtained from Santa Cruz (Santa Cruz, CA, USA). The phospho-IRE1a (pS724) (3881-1) antibody was obtained from Epitomics (Burlingame, CA, USA) and antibodies against β-actin (a2066, 1:5,000) and Flag (F1804, 1:5,000) were purchased from Sigma. The antibodies against Mst1, Mst2, Lats1, phospho-Lats (Ser909), Mob1 and phospho-Mob1 (Thr35) were obtained as described previously [70] . Horseradish peroxidase-conjugated antibodies against rabbit or mouse IgG were obtained from Jackson ImmunoResearch Laboratories (West Grove, PA, USA, 1:3000). The protein bands were visualized using a SuperSignal West Pico Kit (Thermo Fisher Scientific Pierce, IL, USA), according to the manufacturer’s instructions. All the uncropped scans of the most important immunoblottings are included in Supplementary Figs 12–15 . Chromatin immunoprecipitation CHIP assays were performed according to the protocol of the CHIP assay kit (Upstate Biotechnology Inc., NY, USA). Briefly, cells were fixed with 1% formaldehyde for 10 min at room temperature (RT) and then quenched with glycine (125 mM) for 5 min. The fixed cells were washed with PBS containing protease inhibitors and lysed in lysis buffer (pH 8.1) containing 1% SDS, 10 mM EDTA, 50 mM Tris-HCl, and protease inhibitors, for 10 min on ice before the sonication, centrifugation and addition of dilution buffer. One per cent of input was removed and the lysates were immunoprecipitated with 2 μg of rabbit anti-ATF4 antibody (Proteintech Group Inc.), species-matched IgG control antibody or 40 μl of A/G-Sepharose beads for 2 h. Salmon sperm DNA/protein A/G-Sepharose beads were added to the polyclonal ATF4 and IgG control immunoprecipitations for incubation overnight. Immune complexes were washed with low-salt buffer, high-salt buffer, LiCl buffer and twice with TE sequentially before elution in 200 μl of elution buffer (1% SDS, 0.1 M NaHCO 3 ). The elutes were heated at 65 °C for 4 h to reverse the cross-linking and treated with RNase A for 30 min at 37 °C, followed by treatment with proteinase K for 1 h at 45 °C, to remove RNA and protein. DNA was recovered using a QIAGEN PCR purification kit and eluted in 50 μl of QIAGEN EB buffer (QIAGEN, Hilden, Germany). One per cent of input and 10% of the immunoprecipitates were used in PCR analyses using AmpliTaq Gold DNA polymerase (Applied Biosystems, CA, USA) for 35 cycles at 95 °C for 30 s, 51 °C for 30 s, 72 °C for 60 s (after an initial denaturation for 10 min at 95 °C). The primers used for CHIP are shown in Supplementary Table 2 . Flow cytometry assays and quantification Apoptosis assay . Cells were collected by centrifugation at 1,500 r.p.m., washed once in Annxin V binding buffer and incubated with annexin V-APC and DAPI (4′,6-diamidino-2-phenylindole) for 15 min at RT before acquisition on a flow cytometer BD LSRFortessa (BD Biosciences). Flow cytometry data were performed using FlowJo software (Treestar, Ashland, US). ER-Tracker or Mito-Tracker assays . Cultured cells were treated as indicated and the medium was removed from the culture dish. Cells were rinsed with Hank’s balances salt solution, added prewarmed 1 μm ER-Tracker (Molecular Probes, E34250) or 0.5 μm Mito-Tracker (Molecular Probes, M7514) staining solution and incubated for ∼ 30 min at 37 °C/5% CO 2 . The cells were then trypsinized, pelleted by centrifugationand resuspended in Hank’s balances salt solution for flow cytometry analysis. Flow cytometry data were plotted and quantified with median fluorescence intensity using FlowJo software. Intracellular Ca 2+ Measurement . The intracellular Ca 2+ was measured using the Fluo-4 AM Calcium Assay Kit (Invitrogen), according the manufacturer’s protocol. Briefly, cultured cells were trypsinized, washed and incubated with 3 μm Fluo-4 AM for 30 min at 37 °C. After incubation, cells were washed three times with Ca 2+ /Mg 2+ PBS (0.1 mM CaCl 2 and 1 mM MgCl 2 ). The fluorescence in each sample was analysed using the 530/30 filter on the BD LSRFortessa. Baseline calcium levels were recorded for 60 s and were followed by the addition of 2 μm ionomycin (Sigma-Aldrich). After mixing, the samples immediately continued to record for 240 s. Immunofluorescence The cells on coverslips were fixed with 3.7% formaldehyde in PBS at RT for 15 min, rinsed with PBS and then incubated with 0.2% Triton X-100, 0.2% BSA in PBS on ice for 10 min. Following permeabilization, cells were blocked with 0.02% Triton X-100, 5% BSA in PBS at RT for 30 min. The primary antibodies used were as follows: Yap antibody was obtained as described previously (1:200) [23] , Myc-tag (1:250; Santa Cruz sc-40), HA-tag (1:250; Santa Cruz sc-7392) and Flag-tag (1:500; Sigma). The secondary antibodies (1:1,000) including Alexa488-conjugated anti-mouse IgG (A21202), 488-conjugated anti-rabbit IgG (A21206), 555-conjugated anti-mouse IgG (A31570) and 555-conjugated anti-rabbit IgG (A31572) were purchased from Invitrogen. DNA was stained with mounting medium Vectashield (H1200, Vector Laboratories, CA, USA) containing DAPI. All images were collected using a confocal microscope (Zeiss LSM 780; Zeiss, Germany). Quantification of immunofluorescent signals The mean pixel intensities of Yap or PP1 staining were measured using the Zeiss ZEN lite 2012 software (ZEISS). We calculated the ratios of the mean intensity in the nuclei to the mean intensity in the cytoplasm. For each experiment, the values from several representative cells were averaged and presented with the s.d. Similar results were obtained for several independent experiments. To quantify the amount of cytochrome β5-GFP dots, each dot signal was detected by the eye and the area was measured using the Zeiss ZEN lite 2012 software. The dot structures were quantified by two of the authors in a blinded manner. The ratios of the total areas of cytochrome β5-GFP dots to the overall cellular areas are presented as percentages. Immunohistochemistry Tissue was fixed overnight in 10% neutral-buffered formalin and embedded in paraffin for sectioning. Haematoxylin and eosin staining was performed on 5 μm paraffin sections according to common methods. For immunohistochemistry, fixed and paraffin-embedded liver sections were deparaffinized and incubated in citrate buffer at 95 °C for 40 min for antigen retrieval and then incubated overnight at 4 °C with the primary antibodies including anti-mouse Ki67 (Dako, Glostrup, Denmark), anti-Yap, anti-Bip and anti-p-eIF2a (Cell Signaling). After three washes, tissue sections were incubated with biotinylated anti-mouse IgG (Vector Laboratories) for 1 h at RT and then washed three times, after which streptavidin–horseradish peroxidase conjugates (Vector Laboratories) were added and the slides incubated for another 45 min. After another three washes, DAB solution (Vector Laboratories) was added and the slides were counterstained with haematoxylin. TUNEL reactions were initially done as described by the manufacturer, using the Apoptag Peroxidase in Situ Apoptosis Detection Kit (Millipore). Clonogenic assay for the cell-survival experiment Rapidly growing cells were trypsinized and counted with a hemocytometer. Three millilitres of DMEM full medium containing 500 cells was plated in each of the three wells in the six-well plate. The cells were maintained at 37 °C for 7 days to allow the formation of colonies and were then stained with 0.5% crystal violet (Sigma-Aldrich) in absolute methanol. Statistical analysis All data are representative of at least three independent experiments. All statistical analyses were performed using Prism5 (GraphPad). The data are presented as the mean±s.d. and Student’s t test was used for comparisons between two groups. Survival data was analysed using Kaplan–Meier statistical method. The ratio of the relative expression of the indicated proteins from the tumour patients was plotted and applied with the linear regression t -test. A P -value <0.05 was considered statistically significant. In the graphed data *, **, and *** denote P -values of <0.05, 0.01 and 0.001, respectively. Accession codes: RNA-seq data have been deposited in the Gene Expression Omnibus (GEO) database with accession number GSE57654 . How to cite this article: Wu, H. et al . Integration of Hippo signalling and the unfolded protein response to restrain liver overgrowth and tumorigenesis. Nat. Commun. 6:6239 doi: 10.1038/ncomms7239 (2015).